Ferroic nature of magnetic toroidal order Electric dipoles and ferroelectricity violate spatial inversion symmetry, and magnetic dipoles and ferromagnetism break time-inversion symmetry. Breaking both symmetries favours magnetoelectric charge-spin coupling effects of enormous interest, such as multiferroics, skyrmions, polar superconductors, topological insulators or dynamic phenomena such as electromagnons. Extending the rationale, a novel type of ferroic order violating space- and time-inversion symmetry with a single order parameter should exist. This existence is fundamental and the inherent magnetoelectric coupling is technologically interesting. A uniform alignment of magnetic vortices, called ferrotoroidicity, was proposed to represent this state. Here we demonstrate that the magnetic vortex pattern identified in LiCoPO 4 exhibits the indispensable hallmark of such a ferroic state, namely hysteretic poling of ferrotoroidic domains in the conjugate toroidal field, along with a distinction of toroidal from non-toroidal poling effects. This consolidates ferrotoroidicity as fourth form of ferroic order. Presently, three forms of long-range order, all with individual transformation properties under space- and time-inversion, have been demonstrated to be of primary ferroic nature. We distinguish ferromagnetism (+−), ferroelectricity (−+) and ferroelasticity (++), where the first and second sign represent conservation (+) or violation (−) of space- and time-inversion symmetry, respectively. Existence of a fourth form of ferroic order violating space- and time-inversion symmetry (−−) is compelling and has been proposed. The concept of ferrotoroidicity as this ‘missing piece’ is the topic of this work and the ferroic complement to the space- and time-inversion symmetry-breaking phenomena mentioned in the introductory paragraph [1] , [2] , [3] , [4] , [5] , [6] . In general, a toroidal (−−)-like moment is formed by N ≥2 spins per unit cell. In LiCoPO 4 , our reference compound for the following discussion, we have two pairs of spins yielding oppositely oriented toroidal moments of different amplitude so that a net moment T =(0, T y , T z ) survives. A spontaneous uniform alignment of toroidal moments is the basis of a ferrotoroidic state. In refs 7 , 8 , it was shown that the toroidal moment per unit cell, the ‘toroidization’, is a reasonable choice as order parameter. In particular, it does not diverge or depend on the choice of origin for the distance vectors r i . In spite of all this, the concept of ferrotoroidicity as additional form of ferroic order remains questionable because cyclic hysteretic poling between different single-domain states in a conjugate field has never been shown. This reversibility is crucial as exemplified by crystals with regions of opposite optical activity [9] . Since no conjugate field exists that would allow to exert a direct gyrotropic force promoting the crystal towards single-domain optical activity, there is no ‘ferrogyrotropy’. The possibility of toroidal order in crystals has been considered since 1984 (refs 8 , 10 , 11 , 12 , 13 ). A variety of candidate materials were identified by their linear magnetoelectric properties: induction of an electric polarization by a magnetic field ( P i ∝ α ik H k ) and of a magnetization by an electric field ( M k ∝ α ik E i ) [14] , [15] , [16] , [17] . Minimization of the free energy of a system with macroscopic toroidization reveals [7] that the toroidal moment is uniquely related to a magnetoelectric effect according to α ij = ε ijk T k with as the Levi-Civita tensor. An antisymmetric contribution to the magnetoelectric effect thus indicates the presence of a toroidal moment [13] (more on this issue in the Supplementary Discussion ). Just like all ferroelectrics are pyroelectric, but not vice versa, such magnetoelectric response is, however, insufficient for evidencing ferrotoroidicity. For evidencing the ferroic nature of an ordered state, two verifications are obligatory [18] . (i) The existence of domains as regions with different orientation of the order parameter; and (ii) hysteretic orientation of these domains between opposite single-domain states in the conjugate external field, as discussed above. In 2007, the first criterion was fulfilled by relating the domain structure in LiCoPO 4 to ferrotoroidicity [19] . Verification of the more fundamental second criterion and, thus, the ultimate step that could establish ferrotoroidicity as fourth form of ferroic order are still due. Using the analogy to the established types of ferroic order one can specify the properties of the conjugate field required for ferrotoroidic poling, that is, vector-like nature and the simultaneous violation of space- and time-inversion symmetry [8] . A way to generate such a toroidal field S is to apply magnetic and electric fields together and consider S ∝ E × H . A side effect of this approach is that the magnetic and electric fields not only establish the toroidal field S but in addition may also act on the sample on their own or by non-toroidal contributions to the linear magnetoelectric effect [20] . In the maybe closest approach, experiments revealed a sensitivity of the polarized neutron diffraction yield to the signs of simultaneously applied magnetic and electric fields in field-cooling experiments in MnPS 3 and LiFeSi 2 O 6 (refs 21 , 22 ). These results, however, are insufficient for verifying a ferroic state since key aspects such as hysteretic sub-Curie temperature poling of domains and the distinction between toroidal and non-toroidal contributions to the magnetoelectric effect were not shown. In LiCoPO 4 , a toroidal moment was reoriented via a nonlinear magnetic-field effect, that is, not by coupling to the toroidal order parameter [23] . Reports on ferrotoroidic poling are thus virtually non-existent. Here we establish the ferroic nature of toroidal order, using LiCoPO 4 as model case. By laser-optical second-harmonic generation (SHG), we measure the hysteretic response of LiCoPO 4 to a conjugate toroidal field, including the spatially resolved evolution of the domains throughout the poling cycle. We then verify that this response is solely determined by the cooperation of the toroidal-field-establishing magnetic and electric fields and not by either of these fields alone. Most importantly, we separate the toroidal from any non-toroidal contribution to the poling process and find a dominance of the toroidal field. Magneto-crystallographic structure of LiCoPO 4 LiCoPO 4 is chosen as model compound for our experiments because its magnetoelectric properties, its toroidal unit-cell structure and the distribution of its domains have been well characterized [7] , [19] , [23] , [24] , [25] . LiCoPO 4 has the olivine crystal structure and possesses mmm 1′ point symmetry in the paramagnetic state. Below 21.8 K, the Co 2+ magnetic moments form a collinear magnetic order. The resulting point symmetry is 2′ that allows a toroidal moment T =(0, T y , T z ). (Note that one of these vector components was originally denoted as ‘antiferromagnetic’ [19] , a misconception that was corrected later on [7] , [26] .) As Fig. 1a shows, the net toroidal moment in LiCoPO 4 arises as a superposition of two complementary toroidal moments, each generated by N =2 spins. These two contributions to T possess opposite orientation, but a different amplitude, so that they do not compensate and reveal a net moment T ≠0. As detailed in ref. 24 , T z is associated to the loss of the mirror plane m z perpendicular to the z axis. This reduces the point symmetry from mmm 1′ to mmm ′. T y reflects the rotation of the spins by θ =4.6° away from the y axis. This further reduces the magnetic point symmetry to 2′ with respect to the x axis. A calculation [7] reveals T y / T z =sin θ . Thus, T z >> T y , which suggests a much more effective coupling between T z and the toroidal field. In contrast to ref. 19 , we therefore focus on the T z -related subset of domain states, effectively omitting T y and θ , which is like approximating the magnetic point symmetry 2′ by the higher symmetry mmm ′ where T y = θ =0. 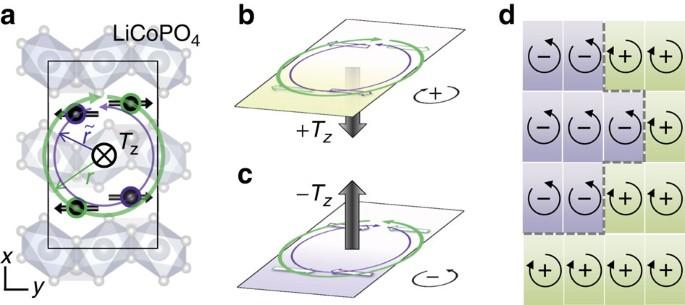Figure 1: Toroidal moment and ferrotoroidic order. (a) Origin of the toroidal momentTzin LiCoPO4shown for the magnetic unit cell (rectangle). Two pairs ofN=2 Co2+spins, highlighted in purple and green, respectively, give opposite contributions toTz. The circumferences associated to the respective pairs show that because of, these two contributions do not cancel. This leads to the net toroidal momentTzparallel to the crystallographiczaxis that breaks the crystallographic mirror symmetry perpendicular to thezaxis. Note that a toroidal momentTy≪Tzis also present. As discussed in the text, however, it is neglected here and shown separately as theSupplementary Fig. 1. (b) Simplified three-dimensional sketch of the toroidal moment ina. (c) Sketch as inb, but for the opposite orientation of the toroidal moment. (d) Periodic continuation of the unit cells sketched inbandcinto a ferrotoroidic crystal with domains in thexyplane. Figure 1: Toroidal moment and ferrotoroidic order. ( a ) Origin of the toroidal moment T z in LiCoPO 4 shown for the magnetic unit cell (rectangle). Two pairs of N =2 Co 2+ spins, highlighted in purple and green, respectively, give opposite contributions to T z . The circumferences associated to the respective pairs show that because of , these two contributions do not cancel. This leads to the net toroidal moment T z parallel to the crystallographic z axis that breaks the crystallographic mirror symmetry perpendicular to the z axis. Note that a toroidal moment T y ≪ T z is also present. As discussed in the text, however, it is neglected here and shown separately as the Supplementary Fig. 1 . ( b ) Simplified three-dimensional sketch of the toroidal moment in a . ( c ) Sketch as in b , but for the opposite orientation of the toroidal moment. ( d ) Periodic continuation of the unit cells sketched in b and c into a ferrotoroidic crystal with domains in the xy plane. Full size image Second-harmonic generation An established probe for imaging domains is SHG, a nonlinear optical process denoting the emission of light at frequency 2 ω from a crystal irradiated with light at frequency ω . This is expressed by the equation , in which E ( ω ) and P (2 ω ) are the electric field components of the incident light and the nonlinear polarization, respectively, with the latter acting as source of the SHG wave of intensity I SHG ∝ | P (2 ω )| 2 (ref. 27 ). The nonlinear susceptibility characterizes the host material. Following the Neumann principle, symmetry determines the set of tensor components χ ijk ≠0. Ferrotoroidic order affects this symmetry and leads to polar, time-non-invariant (‘c-type’) [28] contributions which couple, to the first order, linearly to the order parameter T , so that . Thus, SHG light from opposite ferrotoroidic domain states exhibits a relative 180° phase shift that allows to distinguish these domain states in an interference experiment [29] . In the Methods section, we describe the SHG technology in detail and in the Supplementary Methods , we discuss the time non-invariance and the non-zero components of the SHG tensor (refs 30 , 31 ). 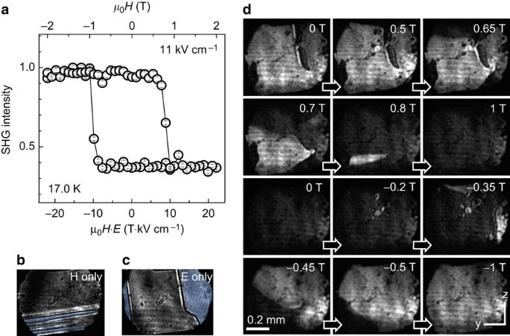Figure 2: Poling and domain structure of a LiCoPO4(100) sample in magnetic and electric fields. (a) SHG intensity at 17.0 K in dependence of a static magnetic fieldμ0Hxtuned between +2 T and −2 T in the presence of a static electric fieldEy=11 kV cm−1. SHG at 2ħω=2.385 eV is emitted from the sample (~χzzz) and superimposed with a SHG reference wave from a quartz plate (~χref) as detailed in the Methods section. Here and in all following figures, error bars indicate the statistical error of the photon count. SHG intensities are arbitrarily scaled with respect to the largest measured value ≡ 1. (b,c) Multi-domain states emerging after cooling the sample in a magnetic or electric field only (b:μ0Hx=7 T,Ey=0;c:Ey=11 kV cm−1,μ0Hx=0). Since contributions fromχrefwere not used in these runs, opposite domains are artificially shaded in different colours. (d) Typical progress of the domain structures of a LiCoPO4(100) sample throughout a magnetic-field-driven hysteresis loop at constant electric field. Images were taken at 17.7 K, 10 kV cm−1, and 2ħω=2.330 eV. (Note that the coercive field is temperature dependent, varying reproducibly by about an order of magnitude between 17.0 and 17.7 K (not shown)). Hysteretic poling Figure 2a shows the response of LiCoPO 4 (100) at 17 K to which a fixed electric field E y =11 kV cm −1 and a tunable magnetic field μ 0 H x are applied. A strikingly pronounced hysteresis is observed in the integrated SHG intensity when cycling the magnetic field in a ±2-T interval. The hysteresis is centred and reveals a coercive field of 0.9 T or 10 T kV cm −1 . We note that even in a field-cooling run through the ordering temperature, a magnetic field ( μ 0 H x =7 T) or an electric field ( E y =11 kV cm −1 ) applied alone leaves the sample in a multi-domain state; Fig. 2b,c . A series of SHG images tracing a hysteresis is shown in Fig. 2d . We see that with the cycling field, the sample alternates between opposite single-domain states of different brightness. In the intermediate multi-domain state domains possess a lateral size in the order of 100 μm. Just like in other ferroic compounds nucleation and growth of domain walls appear to determine the domain reversal. The progressing domain walls, however, do not possess the preferred orientation often imposed by field energy minimization in other ferroics. For the ferrotoroidic order this may be expected, although, because its field energy was calculated to be smaller than that associated to magnetic, electric or elastic order [7] , [8] . Figure 2: Poling and domain structure of a LiCoPO 4 (100) sample in magnetic and electric fields. ( a ) SHG intensity at 17.0 K in dependence of a static magnetic field μ 0 H x tuned between +2 T and −2 T in the presence of a static electric field E y =11 kV cm −1 . SHG at 2 ħω =2.385 eV is emitted from the sample (~ χ zzz ) and superimposed with a SHG reference wave from a quartz plate (~ χ ref ) as detailed in the Methods section. Here and in all following figures, error bars indicate the statistical error of the photon count. SHG intensities are arbitrarily scaled with respect to the largest measured value ≡ 1. ( b , c ) Multi-domain states emerging after cooling the sample in a magnetic or electric field only ( b : μ 0 H x =7 T, E y =0; c : E y =11 kV cm −1 , μ 0 H x =0). Since contributions from χ ref were not used in these runs, opposite domains are artificially shaded in different colours. ( d ) Typical progress of the domain structures of a LiCoPO 4 (100) sample throughout a magnetic-field-driven hysteresis loop at constant electric field. Images were taken at 17.7 K, 10 kV cm −1 , and 2 ħω =2.330 eV. (Note that the coercive field is temperature dependent, varying reproducibly by about an order of magnitude between 17.0 and 17.7 K (not shown)). Full size image In Fig. 3 the relation between the magnetic and the electric field is quantified. In Fig. 3a,b , we see typical hysteresis loops recorded at fixed magnetic and tunable electric field and vice versa. In separate runs, both the sign and the amplitude of the fixed field was varied as presented in Fig. 3c . The result is a spectacular confirmation that solely the product of the magnetic and the electric field determines the shape of the hysteresis loops. In all graphs in Fig. 3c , the single-domain state associated to the low SHG yield is encountered once a field of +0.25 T kV cm −1 is exceeded. In turn, decreasing the field below −0.25 T kV cm −1 leads to the single-domain state associated to the high SHG yield. As a result, all hysteresis loops lie upon one another. As further confirmation, magnetic and electric fields applied alone do not change the multi-domain state ( Fig. 2b,c ). This excludes an interference from nonlinear magnetic- or electric-field effects [23] . 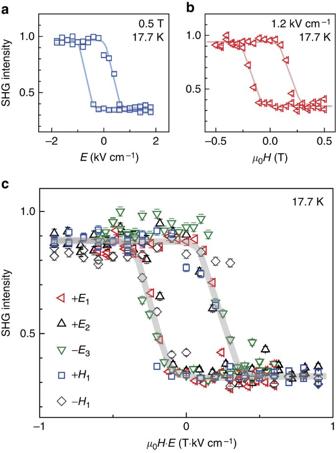Figure 3: Prevalence of the product of magnetic and electric fields in the poling procedure. (a,b) SHG hysteresis loops obtained on LiCoPO4(100) at 17.7 K and 2ħω=2.339 eV under (a) static magnetic fieldHx=+0.5 T and tunable electric fieldEy, and (b) static electric fieldEy=+1.2 kV cm−1and tunable magnetic fieldHx. (c) Various combinations in signs and amplitudes of static and tunable magnetic and electric fields (+E1=+1.2 kV cm−1, +E2=+1.8 kV cm−1, −E3=−1.0 kV/cm, +H1=+0.5 T, −H1=−0.5 T). In all these cases, the coercive field and the domain state are solely determined by the product (Ey·Hx) withμ0|EH|co.=0.25 T kV cm−1as coercive field. Solid lines are guides to the eye. Figure 3: Prevalence of the product of magnetic and electric fields in the poling procedure. ( a , b ) SHG hysteresis loops obtained on LiCoPO 4 (100) at 17.7 K and 2 ħω =2.339 eV under ( a ) static magnetic field H x =+0.5 T and tunable electric field E y , and ( b ) static electric field E y =+1.2 kV cm −1 and tunable magnetic field H x . ( c ) Various combinations in signs and amplitudes of static and tunable magnetic and electric fields (+ E 1 =+1.2 kV cm −1 , + E 2 =+1.8 kV cm −1 , − E 3 =−1.0 kV/cm, + H 1 =+0.5 T, − H 1 =−0.5 T). In all these cases, the coercive field and the domain state are solely determined by the product ( E y · H x ) with μ 0 | EH | co. =0.25 T kV cm −1 as coercive field. Solid lines are guides to the eye. Full size image Toroidal and non-toroidal poling In the final step, we need to distinguish ferrotoroidic from non-ferrotoroidic contributions to the magnetoelectric poling process. Only the antisymmetric product of magnetic and electric fields establishes the toroidal field [8] , which may thus be represented by the coefficients . Any symmetric contributions ( ) relate to conventional non-toroidal magnetoelectric poling such as in Cr 2 O 3 (ref. 32 ) and need to be separated. The insets to Fig. 4a,b show two field configurations that allow us to distinguish toroidal and non-toroidal contributions. We apply magnetic and electric fields ( E x H y ∓ E y H x )/2 so that we couple to the components α xy ∓ α yx . The associations and are obvious. Exemplary hysteresis loops obtained on a LiCoPO 4 (001) sample are shown in Fig. 4 . Note that Fig. 4a shows the first example of purely toroidal hysteretic poling of a ferrotoroidic domain structure. The non-toroidal poling, too, can drive the sample into a single-domain state ( Fig. 4b ), but here the coercive field is a different one. With loops as in Fig. 4 , the ratio of the coercive fields was determined in >20 runs performed at three different voltages with the result shown in Fig. 4c . We find , which is a first quantitative indication that the toroidal and the non-toroidal poling fields indeed couple to different material properties. 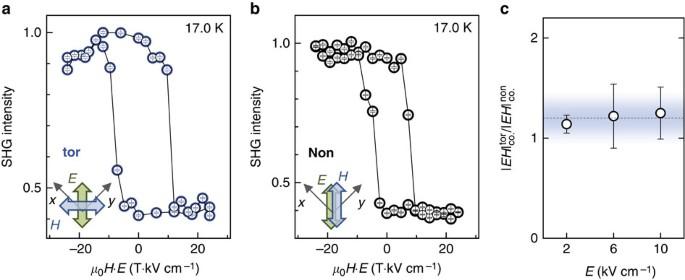Figure 4: Distinction between ferrotoroidic and non-ferrotoroidic contributions to the magnetoelectric poling procedure. (a) Purely toroidal hysteresis loop. (b) Non-toroidal hysteresis loop.aandbwere obtained at 2ħω=2.330 eV and 17.0 K on LiCoPO4(001) withE=12 kV cm−1. The respective experimental field configurations are sketched as insets. (c) Ratio of the coercive fields obtained by toroidal and non-toroidal poling at different electric fields. Error bars result from >20 consecutive runs. Figure 4: Distinction between ferrotoroidic and non-ferrotoroidic contributions to the magnetoelectric poling procedure. ( a ) Purely toroidal hysteresis loop. ( b ) Non-toroidal hysteresis loop. a and b were obtained at 2 ħω =2.330 eV and 17.0 K on LiCoPO 4 (001) with E =12 kV cm −1 . The respective experimental field configurations are sketched as insets. ( c ) Ratio of the coercive fields obtained by toroidal and non-toroidal poling at different electric fields. Error bars result from >20 consecutive runs. Full size image From literature it is known [25] that, almost independent of temperature, α yx =2 α xy , which leads to . If the toroidal poling were as effective as the non-toroidal poling in terms of the field energy that is required to switch the LiCoPO 4 sample to a single-domain state, we would expect a ratio of the coercive fields (to compensate for γ α =1/3). The strikingly different experimental value of 1.21 shows that the toroidal field is much more effective in promoting the ferrotoroidic single-domain state. Apparently, the ferrotoroidic and the non-ferrotoroidic contributions to the magnetoelectric field product connect to different types of mechanisms pinning the domain walls and thereby determining the width of the hysteresis. In summary, our demonstration of hysteretic poling of ferrotoroidic domains in LiCoPO 4 in the conjugate toroidal field is a strong argument in favour of regarding ferrotoroidicity as primary ferroic order on a level with ferromagnetism, ferroelectricity and ferroelasticity. The toroidal field was generated magnetoelectrically with simultaneously applied static magnetic and electric fields. Using different setups, we explicitly distinguished its action from interfering action of the non-toroidal magnetoelectric effect. In addition, spatially resolved images of the progressing ferrotoroidic domain structure throughout a hysteretic poling cycle were recorded. With ferrotoroidicity as fourth form of primary ferroic order, we now have one type of ferroic order for each of the four possible sets of eigenvalues (++, +−, −+ and −−) of the space- and time-inversion operations. Thus, aside from the value of ferrotoroidic materials as compounds inherently providing the coupling of an electric voltage to a magnetization, a fundamental balance of symmetries is achieved by establishing ferrotoroidicity as the previously void space- and time-inversion-antisymmetric ferroic state. It is, however, intriguing that ferrotoroidicity, ferromagnetism and ferroelectricity are characterized by vectors, whereas ferroelasticity as space- and time-inversion-symmetric ferroic state is associated to a rank-two tensor. A possible way to remedy this is the introduction of electrotoroidal order in which the vortex of magnetic moments is replaced by a vortex of electric dipoles. Such kind of order would be characterized by a space- and time-inversion-symmetric vector. So far, electric-dipole vortices have only been observed as a result of geometric confinement, but not in relation to long-range order [33] , [34] . This might pose an interesting challenge to further exploration of the phenomenon of spontaneous long-range order in condensed matter systems. SHG tensor components A symmetry analysis of the magnetic point groups 2′ ( T z , T y , θ ≠0) and mmm ′ ( T z ≠0; T y , θ =0) with x and z as 2′ axis and m ′ plane, respectively, shows that domain states according to the component T z of the toroidal vector are accessible by the polar, time-non-invariant (‘c-type’) SHG susceptibilities χ zzz , χ zxx , χ xxz , χ zyy , χ yyz (ref. 28 ). In the index triplet χ ijk , the first index denotes the polarization of the emitted SHG wave and the latter two indices denote the polarization of the two photons from the incident fundamental light wave. All the listed components have been observed and their emergence along with the toroidal structure in Fig. 1a and Supplementary Fig. 1 confirms their coupling to this structure [35] . At the photon energies used in the present experiment, the SHG yield from T y is at least two orders of magnitude smaller than that from T z and can thus be neglected. In the Supplementary Methods , this is further discussed along with the derivation of the transformation properties and non-zero components of the SHG tensor. Introductions to SHG on ordered magnetic moments are given in refs 30 , 31 . Samples and experimental setup LiCoPO 4 bulk samples were cut perpendicular to the (100) or the (001) axis and polished with an aqueous colloidal silica slurry. The samples had lateral dimensions of 1–3 mm and a thickness of ~100 μm. They were mounted in a liquid-helium-cooled variable-temperature cryostat generating magnetic fields of up to 7 T. The cryostat was equipped with a non-commercial sample holder for applying a static voltage of up to 6 kV. A transmission setup described in detail in refs 29 , 31 was used. The LiCoPO 4 samples were excited with light pulses of 3 ns and ~1 mJ emitted from an optical parametric oscillator. Maximum SHG yield is obtained between 2.30 and 2.40 eV so that 1.15–1.20 eV was chosen as photon energy of the incident light [19] . For the (100)-oriented samples, the light was incident along the x axis and the T z -related toroidal order was probed by χ zzz . The laser light was transmitted through the sample, mounted in a cryostat and through a quartz crystal placed behind the cryostat. The SHG light was emitted from the sample and the quartz was projected onto a liquid-nitrogen-cooled digital camera by a telephoto lens. On the camera, the SHG light from the sample (~ χ zzz ) and from the quartz (~ χ ref ) interfered so that opposite T z -related domain states appeared as bright and dark regions, respectively, because of the 180° SHG phase shift between the domain states that is explained in the main text [29] . For the (001)-oriented samples, the cryostat was slightly rotated so that the incident light included an angle of ~15° with the z axis. Because of this rotation, the χ zxx component became accessible for probing the T z -related toroidal order. Furthermore, SHG components ~ χ ref not coupling to the magnetic order could be excited in the LiCoPO 4 in this configuration so that the quartz plate was removed from the setup. How to cite this article : Zimmermann, A.S. et al . Ferroic nature of magnetic toroidal order. Nat. Commun. 5:4796 doi: 10.1038/ncomms5796 (2014).